Streptomycin potency is dependent on MscL channel expression The antibiotic streptomycin is widely used in the treatment of microbial infections. The primary mechanism of action is inhibition of translation by binding to the ribosome, but how it enters the bacterial cell is unclear. Early in the study of this antibiotic, a mysterious streptomycin-induced potassium efflux preceding any decrease in viability was observed; it was speculated that this changed the electrochemical gradient such that streptomycin better accessed the cytoplasm. Here we use a high-throughput screen to search for compounds targeting the mechanosensitive channel of large conductance (MscL) and find dihydrostreptomycin among the ‘hits’. Furthermore, we find that MscL is not only necessary for the previously described streptomycin-induced potassium efflux, but also directly increases MscL activity in electrophysiological studies. The data suggest that gating MscL is a novel mode of action of dihydrostreptomycin, and that MscL’s large pore may provide a mechanism for cell entry. Streptomycin was the first antibiotic to be discovered in the aminoglycoside class and is derived from an actinobacterium of the Streptomyces genus [1] . It is widely used in the treatment of serious bacterial infections caused by both Gram-negative and Gram-positive bacteria, including tuberculosis, endocardial and meningeal infections and the plague. Although it is known that the primary mechanism of action of streptomycin is through inhibition of protein synthesis by binding the ribosome, the mechanism of entry to the bacterial cell is not yet clear. Mechanosensitive channel of large conductance (MscL) is a highly conserved bacterial mechanosensitive channel that directly senses tension in the membrane [2] . The physiological role of MscL is that of an emergency release valve that gates upon an acute drop in the osmolarity of the environment (hypo-osmotic downshock) [3] . Under hypo-osmotic stress, water enters the bacterial cell causing it to swell, thus increasing tension in the membrane; MscL gates in response to this tension forming a large pore of about 30 Å [4] , thus allowing for the rapid release of solutes and saving the cell from lysis. Because of the large pore size, MscL gating is tightly regulated; expression of a mis-gating MscL channel, which opens at lower than normal tensions, causes slow bacterial growth or even cell death [5] . Bacterial mechanosensitive channels have been proposed as ideal drug targets owing to their important role in the physiology of bacteria and the lack of identified homologues in higher organisms [6] . We therefore performed a high-throughput screen (HTS) searching for compounds that will inhibit bacterial growth in a MscL-dependent manner. Interestingly, among the hits we found four known antibiotics, among them the widely used aminoglycosides antibiotics streptomycin and spectinomycin. Here we show that the potency of streptomycin is dependent on MscL expression in growth and viability experiments in vivo. We also provide evidence of the direct modulation of MscL channel activity by dihydrostreptomycin in patch clamp experiments in vitro . The involvement of MscL in the pathway of streptomycin action suggests not only a novel mechanism for how this bulky and highly polar molecule obtains access to the cell at low concentrations, but also new tools to modulate the potency of already known and potential antibiotics. HTS reveals an MscL-dependent effect of known antibiotics Under the hypothesis that MscL could serve as an antibiotic target, we performed a HTS of the UT Southwestern small-molecule library (~230,000 compound) in search of MscL agonists, looking for compounds that would gate the channel and thus inhibit Escherichia coli bacterial growth in a MscL-dependent manner (see Methods for HTS details). Briefly, we used the E. coli MJF612 strain (Frag1 Δ mscL , Δ mscS , Δ mscK , Δ ybdG ) [7] expressing K55T E. coli MscL (K55T MscL), a mild gain-of-function mutant, and had bacterial growth as an output, measured as the optical density of the cultures at 595 nm (OD 595 ). Surprisingly, four known antibiotics were identified as potential candidates for MscL-specific decreased bacterial growth: dihydrostreptomycin, spectinomycin, viomycin and nifuroxazide. However, the primary mechanisms of action of these antibiotics are already known, with streptomycin, spectinomycin and viomycin affecting protein synthesis [8] , [9] , [10] and nifuroxazide inhibiting dehydrogenase enzyme activity and causing DNA damage [11] , [12] . Growth inhibition assays of these known antibiotics were performed using the same strain and mutant, K55T MscL, used in the original HTS [5] . For all four of the drugs, a concentration was easily found at which cells expressing K55T MscL, but not those containing empty plasmid, showed an antibiotic-dependent decreased growth. We then used this antibiotic concentration and assayed growth of the same cells expressing wild-type (WT) Eco-MscL as well as MscL orthologues from the Gram-positive Bacillus subtilis and Staphylococcus aureus . An unrelated E. coli mechanosensitive channel that also detects membrane tension, MscS, was included to determine drug specificity for MscL. The results of these experiments are summarized in Fig. 1 . The aminoglycoside antibiotics dihydrostreptomycin and spectinomycin showed the clearest MscL dependence, affecting the growth of cells expressing all three MscL orthologues significantly more than the empty vector or MscS-expressing cells. Viomycin also inhibited the growth of cells expressing the MscS channel and the orthologues, but not the WT Eco-MscL. Finally, although nifuroxazide had a milder effect on growth inhibition, it also showed a significant dependence on MscS as well as MscL channel expression. The observation that viomycin and nifuroxazide are MscS- and MscL-expression dependent in their potency suggests that they are non-specific activators of membrane tension-gated channels. They most likely work by intercalating into and adding tension within the cell plasma membrane, consistent with the finding that amphipaths, including lysophosphatidylcholine, could gate these channels [13] , [14] . On the other hand, the aminoglycoside antibiotics dihydrostreptomycin and spectinomycin appeared to be specifically MscL-dependent, and thus are likely to have direct influences on the MscL channel, with dihydrostreptomycin being more potent. We therefore continued our analysis of dihydrostreptomycin, which seemed the most tractable system. 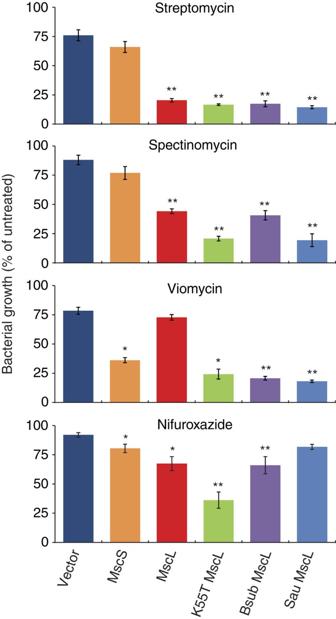Figure 1: MscL-dependent inhibition of bacterial growth by known antibiotic agents. Effects of antibiotics on the growth of bacteria hosting an empty vector (dark blue) or expressingE. coliMscS (orange),E. coliMscL (red), K55T MscL (green),B. subtilus(purple) andS. aureusMscL(light blue). The bars represent the growth of bacteria in the presence of 6.5 μM dihydrostreptomycin, 100 μM spectinomycin, 80 μM viomycin or 7.5 μM nifuroxazide, expressed as the percentage of the untreated sample ((OD600treated/OD600untreated) × 100). Error bars represent s.e.m. (n=4–5 independent experiments). *P<0.0075, **P<0.00005, Student’st-test unpaired versus vector. Figure 1: MscL-dependent inhibition of bacterial growth by known antibiotic agents. Effects of antibiotics on the growth of bacteria hosting an empty vector (dark blue) or expressing E. coli MscS (orange), E. coli MscL (red), K55T MscL (green), B. subtilus (purple) and S. aureus MscL(light blue). The bars represent the growth of bacteria in the presence of 6.5 μM dihydrostreptomycin, 100 μM spectinomycin, 80 μM viomycin or 7.5 μM nifuroxazide, expressed as the percentage of the untreated sample ((OD 600 treated/OD 600 untreated) × 100). Error bars represent s.e.m. ( n =4–5 independent experiments). * P <0.0075, ** P <0.00005, Student’s t -test unpaired versus vector. Full size image Streptomycin potency is MscL dependent in vivo A full concentration curve comparing growth inhibition by dihydrostreptomycin of cells expressing MscL or an empty plasmid clearly shows that MscL-expressing cells are susceptible to lower concentrations of the antibiotic ( Fig. 2a ). Furthermore, when comparing the effects of dihydrostreptomycin between a strain that expresses endogenous levels of MscL (MJF451) with another strain null for MscL (MJF455), we still observe a higher growth inhibition by streptomycin in the bacteria endogenously expressing MscL ( Supplementary Fig. 1a ). To verify that growth inhibition, measured as OD 600 , reflected the changes in bacterial viability and not just altered bacteria cell shape or size, we performed viability experiments on agar plates containing different concentrations of dihydrostreptomycin. As shown in Fig. 2b , at 3 or 4 μM drug, viability of bacteria expressing WT and K55T MscL was one to three orders of magnitude lower than the viability of cells carrying empty vector or expressing the other major mechanosensitive channel, MscS; note that all cells showed decreased viability at higher concentrations of dihydrostreptomycin ( Supplementary Fig. 1b ), consistent with the hypothesis that MscL increases potency, but is not the primary mechanism of action of the drug. These results are in good agreement with the observed MscL-dependent growth inhibition in liquid culture growth experiments ( Fig. 1 ), demonstrating that MscL expression increases bacterial susceptibility to dihydrostreptomycin. 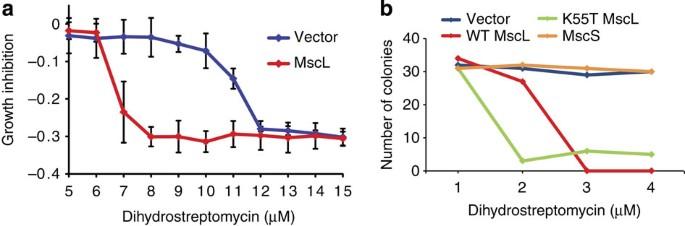Figure 2: MscL-dependent susceptibility to dihydrostreptomycin. (a) Growth inhibition of liquid cultures ofE. colibacteria hosting an empty vector (dark blue) or expressingE. coliMscL (red) were grown at different dihydrostreptomycin concentrations. The data are expressed as the reduction in growth, measured at OD (600), of the treated cultures compared with the untreated cultures. Error bars reflect s.e.m. (n=3–4 independent experiments). (b) The viability of bacteria carrying an empty vector (blue) or expressingE. coliMscL (red),E. coliMscS (orange) or K55T MscL (green) was measured in agar plates with different concentrations of dihydrostreptomycin. The number of viable colonies as a function of the antibiotic concentration is shown for one representative experiment. Figure 2: MscL-dependent susceptibility to dihydrostreptomycin. ( a ) Growth inhibition of liquid cultures of E. coli bacteria hosting an empty vector (dark blue) or expressing E. coli MscL (red) were grown at different dihydrostreptomycin concentrations. The data are expressed as the reduction in growth, measured at OD (600), of the treated cultures compared with the untreated cultures. Error bars reflect s.e.m. ( n =3–4 independent experiments). ( b ) The viability of bacteria carrying an empty vector (blue) or expressing E. coli MscL (red), E. coli MscS (orange) or K55T MscL (green) was measured in agar plates with different concentrations of dihydrostreptomycin. The number of viable colonies as a function of the antibiotic concentration is shown for one representative experiment. Full size image Streptomycin-induced K + flux is MscL dependent Early studies trying to determine the mechanism of action of streptomycin found that, upon drug treatment a rapid flux of K + out of the cell was observed prior to any decrease in viability [15] . Moreover, the same group describes a significant increase in streptomycin uptake if the bacteria are pre-diluted in a lower osmolarity media (hypo-osmotic shock) prior to streptomycin incubation [16] . Potassium is one of the major osmoprotectants, reaching several 100 mM in the cytoplasm, and can be fluxed by MscL from the cytoplasm in response to osmotic downshock [17] , [18] . Under the hypothesis that the observed K + -flux could be due to MscL activation by streptomycin, we compared the K + -flux induced by dihydrostreptomycin in bacterial cells with or without MscL expression. We measured the K + remaining in the cells [17] , as well as viability, after different incubation times with dihydrostreptomycin. Briefly, cultures at approximately OD 600 =0.2 were induced for 1 h at 37 °C, then split in two: mock (no drug added) and with dihydrostreptomycin. The final OD 600 was taken and the amount of cells to be used was calculated, adjusting for OD. Approximately 1–1.5 ml of the cultures were then passed through a 0.45-μm filter and washed, then dried as described in Methods. Three ml of double-distilled water were added to each filter, and K + levels were read using a flame photometer after a standard curve was established. Control values from four independent experiments were 131±3 μM. As shown in Fig. 3a , a K + -flux was observed after treatment of MscL-expressing bacteria; note that at 20 min there is a significant K + flux, but no measurable decrease in viability ( Fig. 3a ). No significant flux or decrease in viability was observed in cells not expressing MscL at this concentration of drug ( Fig. 3b ). Note that the dihydrostreptomycin concentration used in these experiments (82 μM) is higher than that used in the growth inhibition experiments, because a higher osmolarity media was used for the cells to accumulate K + ; as previously described, higher streptomycin concentrations are needed to achieve the same effect in high-osmolarity media [19] . Note that even at 40 min, little viability loss is noted in Fig. 3b , where MscL is not expressed. We therefor tested this strain at a higher streptomycin concentration at which about a 50% decrease in viability is observed at 40 min. However, even at this concentration, only modest streptomycin-induced K + -flux is observed, and only after the decreases in viability occurred ( Fig. 3c ). These results strongly suggest that the streptomycin-induced K + -flux is due to MscL activation. 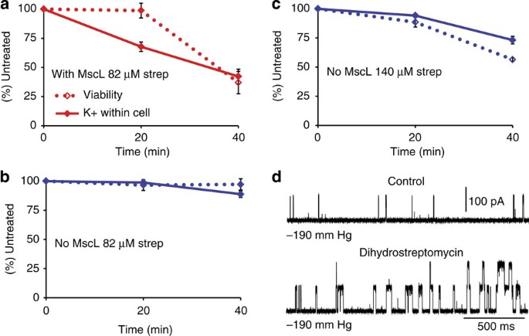Figure 3: Modulation of MscL channel activity by streptomycin. (a) The graph shows the percentage of potassium remaining in the a MscL null bacterial strain expressingE. coliMscLin trans(red solid line). Cell viability after 20 or 40 min of incubation with 82 μM dihydrostreptomycin is also shown (red dotted line). Values are expressed as a percentage of values from the untreated cells. Error bars reflect s.e.m. (n=4 independent experiments). (b) The graph shows the percentage of potassium remaining in a MscL null bacterial strain hosting the empty plasmid, pB10b, with no MscL insert (blue solid line). Cell viability after 20 or 40 min of incubation with 82 μM dihydrostreptomycin is also shown (blue dotted line). Values are expressed as a percentage of values from the untreated cells. Error bars reflect s.e.m. (n=4 independent experiments). (c) The graph shows the percentage of potassium remaining in a MscL null bacterial strain hosting the empty plasmid, pB10b, with no MscL insert (blue solid line), at a higher concentration of streptomycin where decreases in viability could be observed. Cell viability after 20 or 40 min of incubation with 140 μM dihydrostreptomycin is also shown (blue dotted line). Values are expressed as a percentage of values from the untreated cells. Error bars reflect s.e.m. (n=4 independent experiments). (d) Single-channel recordings from patch clamp experiments in native bacterial membranes. The current traces show the activity of K55T MscL held at a potential of −20 mV and a negative pressure of −190 mm Hg, before and after treatment with 50 μM dihydrostreptomycin. Figure 3: Modulation of MscL channel activity by streptomycin. ( a ) The graph shows the percentage of potassium remaining in the a MscL null bacterial strain expressing E. coli MscL in trans (red solid line). Cell viability after 20 or 40 min of incubation with 82 μM dihydrostreptomycin is also shown (red dotted line). Values are expressed as a percentage of values from the untreated cells. Error bars reflect s.e.m. ( n =4 independent experiments). ( b ) The graph shows the percentage of potassium remaining in a MscL null bacterial strain hosting the empty plasmid, pB10b, with no MscL insert (blue solid line). Cell viability after 20 or 40 min of incubation with 82 μM dihydrostreptomycin is also shown (blue dotted line). Values are expressed as a percentage of values from the untreated cells. Error bars reflect s.e.m. ( n =4 independent experiments). ( c ) The graph shows the percentage of potassium remaining in a MscL null bacterial strain hosting the empty plasmid, pB10b, with no MscL insert (blue solid line), at a higher concentration of streptomycin where decreases in viability could be observed. Cell viability after 20 or 40 min of incubation with 140 μM dihydrostreptomycin is also shown (blue dotted line). Values are expressed as a percentage of values from the untreated cells. Error bars reflect s.e.m. ( n =4 independent experiments). ( d ) Single-channel recordings from patch clamp experiments in native bacterial membranes. The current traces show the activity of K55T MscL held at a potential of −20 mV and a negative pressure of −190 mm Hg, before and after treatment with 50 μM dihydrostreptomycin. Full size image Streptomycin also induces a MscL-dependent glutamate flux When MscL gates, K + is not the only molecule jettisoned from the cell, several osmolytes have also been proposed to go through this channel. One of these is glutamate [20] , whose synthesis is increased upon exposure to high osmolarity [21] , [22] , and whose negative charge is thought to serve as a counter ion for K + . We therefore used the dihydrostreptomycin concentrations above and tested to see if glutamate was also fluxed from the cell in the 20-min timescale in which K + is seen to flux (see Fig. 3a–c ). Briefly, cultures at approximately OD 600 =0.2 were induced for 1 h at 37 °C, then split in two: mock (no drug added) and with dihydrostreptomycin added. The final OD 600 of the cultures was recorded and 15 ml of each sample was pelleted, the supernatant removed and immediately frozen down to −80 °C. Samples were resuspended, adjusting volume for final OD 600 . Glutamate measurements were performed as described in Methods, and control values from three independent experiments was 260±20 μM. While there was no significant loss of glutamate from cells not expressing MscL, 52% of the glutamate was lost from cells expressing it ( Fig. 4 ). Hence, it appears that streptomycin activation of MscL leads not only to the previously reported flux of K + prior to decreases in viability, but also leads to efflux of at least one other osmoprotectant: glutamate. 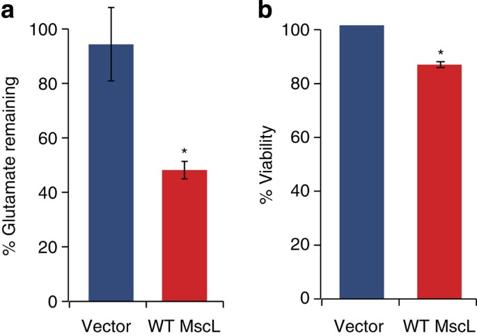Figure 4: Streptomycin induces a MscL-dependent glutamate flux. (a) The flux of glutamate fromE. colibacteria expressing an empty vector or MscL was measured as the percentage of glutamate remaining in the bacterial cells after 20 min of incubation with 82 μM dihydrostreptomycin. Error bars reflect s.e.m. (n=3 independent experiments). (b) The viability of the bacterial cells was measured after the same treatment and graphed as a percentage viability of the untreated samples. Error bars reflect s.e.m. *P<0.021, Student’st-test treated versus untreated paired,n=3. Figure 4: Streptomycin induces a MscL-dependent glutamate flux. ( a ) The flux of glutamate from E. coli bacteria expressing an empty vector or MscL was measured as the percentage of glutamate remaining in the bacterial cells after 20 min of incubation with 82 μM dihydrostreptomycin. Error bars reflect s.e.m. ( n =3 independent experiments). ( b ) The viability of the bacterial cells was measured after the same treatment and graphed as a percentage viability of the untreated samples. Error bars reflect s.e.m. * P <0.021, Student’s t -test treated versus untreated paired, n =3. Full size image Streptomycin modulates MscL activity in patch clamp Finally, we directly assessed the effects of these antibiotics on MscL channel activity in patch clamp. Briefly, we used the MJF612 strain expressing the K55T MscL mutant in trans to make the giant spheroplast preparation, which allows analysis within native bacterial membranes [23] . We applied the drugs in the pipette, which reflects the periplasmic side of the channels, using the back-filled pipette method as previously performed [24] and described in the Methods section. This method allows for the assessment of channel activity within the same patch before and after drug exposure. As shown in Fig. 3d , the presence of the antibiotics has significant effect in channel open probability ( P o treated/untreated 11.9±3.7; P <0.002, Student’s t -test dihydrostreptomycin versus control unpaired n ≥3, n being the number of independent patches before and after treatment). Consistently, a reduction in the pressure required to gate the channels was also observed (pressure threshold treated/untreated 0.85±0.07 P <0.03 Student’s t -test dihydrostreptomycin versus control unpaired n ≥4). No increases in P o or reduction in pressure were observed in MscL untreated patches or in the activity of the unrelated mechanosensitive channel MscS ( Supplementary Fig. 2 ). Similar increases in sensitivity of MscL mutants have previously been associated with potassium flux and slowed growth and decreases in viability [5] . The effects observed here on the channel sensitivity in patch clamp may be an underestimation owing to the difference in membrane potential (approximately −180 mV intact cell versus −20 mV patch), given that dihydrostreptomycin is positively charged and a more negative membrane potential might favour interactions with the MscL channel at the membrane; note also that there is precedence for an increase in open probability at higher membrane potentials [17] . In sum, these experiments demonstrate that dihydrostreptomycin increases MscL channel activity. Here we present a novel mechanism for a known antibiotic: the specific activation of the mechanosensitive channel MscL. Although other studies have suggested that some compounds modulate MscL activity, specificity has never been demonstrated. For the bacterial toxin sublancin 168 (ref. 25) [25] , a lantibiotic, a MscL-dependent viability of B. subtilis and S. aureus bacteria in vivo was observed, but no electrophysiological studies were performed, nor was there an assessment of the role MscS may play; hence, it is not clear whether this lantibiotic acts directly or specifically with MscL. Another group of antimicrobial agents, parabens, as well as the spider toxin GsMTx4, have been reported to affect MscL as assayed by patch clamp, but no in vivo studies have determined any MscL-dependent effects for either class of compounds, and in patch experiments, they also influence MscS, suggesting that they work through an indirect mechanism involving the lipid membrane [26] , [27] , [28] . Thus, there has previously been no compound shown to directly and specifically influence MscL gating. Here we demonstrate that dihydrostreptomycin directly induces MscL activity, thus increasing the potency of the drug. In addition, this appears to be specific because, unlike viomycin and nifuroxazide, no difference in potency was observed upon MscS expression. We therefore propose a model for how MscL increases the potency of streptomycin that is consistent with previous findings as well as the data presented here ( Fig. 5 ). Initially, streptomycin interacts with MscL and activates it, thus leading to an outward flux of K + . The present data cannot exclude the possibility of streptomycin acting through another protein associated with the MscL channel, although no such interactions of MscL have ever been reported, thus a direct interaction would be the simplest data interpretation. This occurs within 20 min, but is not correlated with a detectable decrease in viability. According to early studies by Busse et al. [29] , the streptomycin-induced K + flux does not lead to a decrease in the steep bacterial membrane potential (ca −165 mV), instead a slight hyperpolarization is observed. This hyperpolarization is not as great as one might expect if only K + was lost from the cell, so the authors speculated that anions may also flux from the cytoplasm. This finding is consistent with our results demonstrating a loss of glutamate, as well as K + , from the cell prior to any loss in viability. The slight hyperpolarization causes an enhanced electrochemical potential for the entrance to the cell of the positively charged streptomycin. Molecular-sieving experiments have previously demonstrated that compounds up to 30 Å can go through the MscL pore [4] . While the resulting decrease in viability could be solely due the channel opening and the loss of solutes, streptomycin, about 10 Å in diameter, is well within this 30-Å size, making it likely that it would easily pass through the channel. Its positive charge would give it a large electrochemical gradient. Thus, the open MscL channel would be a pathway for streptomycin to enter the cell cytoplasm. Perhaps it is this enhanced transport through MscL that is solely responsible for the increase in potency that is observed. However, because streptomycin is still effective when MscL is not expressed, albeit requiring higher concentrations, there must also be alternative pathways to the cytoplasm. Regardless, the observation that spectinomycin also shows an increase in potency when MscL is expressed ( Fig. 1 ) demonstrates that this is not specific for streptomycin, but may be a mechanism common among aminoglycoside antibiotics. Given the finding that MscL activation increases drug potency and may increase the efficiency of a drug entering the bacterial cell, it seems likely that an agonist to MscL could be used as an adjuvant for other known or potential antibiotics to increase their efficacy. 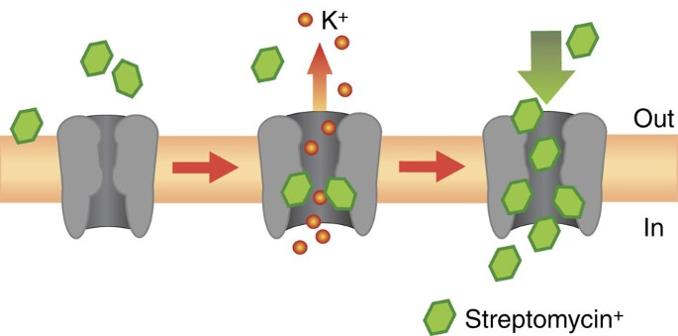Figure 5: Working model for streptomycin–MscL interactions. The model depicts the MscL channel in the lipid membrane, in a series of events starting on the left. A first interaction between streptomycin and the bacteria occurs, leading to the activation of MscL, which allows a K+-flux from the cell. This occurs prior to any decrease in viability. The open MscL pore could serve as a pathway for streptomycin into the cell cytoplasm. It is by this mechanism that MscL expression increases the potency of the drug. Figure 5: Working model for streptomycin–MscL interactions. The model depicts the MscL channel in the lipid membrane, in a series of events starting on the left. A first interaction between streptomycin and the bacteria occurs, leading to the activation of MscL, which allows a K + -flux from the cell. This occurs prior to any decrease in viability. The open MscL pore could serve as a pathway for streptomycin into the cell cytoplasm. It is by this mechanism that MscL expression increases the potency of the drug. Full size image Stains and cell growth Constructs were inserted in the pB10d expression vector [5] , [24] , [30] , [31] and the E. coli strain MJF612 (Frag1 Δ mscL ::cm, Δ mscS , Δ mscK ::kan,Δ ybdG ::aprΔ) [7] was used as a host for all experiments. Unless stated otherwise, cells were grown in citrate-phosphate-defined medium (CphM) consisting of (per liter: 8.57 g of Na 2 HPO 4 , 0.87 g of K 2 HPO 4 , 1.34 g of citric acid, 1.0 g of NH 4 SO 4 , 0.001 g of thiamine, 0.1 g of Mg 2 SO 4 .7H 2 0, 0.002 g of (NH 4 ) 2 SO 4 .FeSO 4 .6H 2 O) plus 1 mM ampicillin. HTS We performed a very simple HTS with bacterial growth as an output measured as the optical density of the cultures at 595 nm (OD 595 ). We tested a total of ~230,000 compounds in the UT Southwestern institutional library and looked for compounds that inhibited bacterial growth ( Z -score<−3) Z -score=(data point value−mean)/s.d. The E. coli strain MJF612 was used as a host for the K55T MscL mutant expressed in trans [5] in pB10d expression vector. The positive control consisted of bacteria expressing the G26C MscL mutant in trans treated with 2 mM MTSET + (Toronto Research Chemicals, Toronto, ON, Canada), which opens MscL and causes severe growth inhibition [32] , [33] . This control was present in every assay plate (column 1). The assay had a Z -prime value >0.75 (ref. 34) [34] . Briefly, overnight cultures grown in CphM were diluted 1:200 in chilled (4 °C) media and kept in ice until loading into plates. The assay was performed in clear 384-well polystyrene plates with a flat bottom, non-treated and sterile (Greiner Bio One, Monroe, NC, USA). Before loading the plates (75 μl per well), cultures were induced with 1 mM isopropyl β- D -1-thiogalactoside (IPTG), and cells expressing G26C MscL were treated with 2 mM MTSET + . The compounds (dissolved in neat dimethyl sulphoxide (DMSO)) were added to a 10-μM final concentration to columns 3–22 of each assay plate, the lids were added, the plates were wrapped in foil and incubated for 14–16 h in a shaker at 37 °C, shaking at 110 r.p.m. Plates were then read at 595 nm. Our primary HTS consisted in a simple assay measuring the growth of bacteria using OD 595 as an output. In this series of experiments, we used the E. coli strain MJF612 that lacks the four major mechanosensitive channels, expressing a very mild MscL mutant expressed in trans , K55T. This mutant was chosen because it is slightly more sensitive to pressure, has only a slightly retarded growth, is not located within the pore and has similar channel kinetics to WT MscL [5] . After normalization of absorbance values to the median of the DMSO controls (columns 2 and 23 of each 384-well assay plate) using GeneData’s Screener analysis software (Assay Analyzer v.10), compounds that inhibited bacterial growth were selected ( Z -score<−3) with a final hit rate of just <1%. After filtering for redundancy, 1,600 compounds were cherry-picked and retested in the primary assay at 10 μM in triplicate. These compounds were also tested in a similar secondary screen that measured the effect of the drugs in cells carrying empty plasmid. This secondary screen was used as a selectivity screen, so the positive hits that inhibited growth of these bacteria lacking MscL were discarded as non-specific. Stationary growth experiments E. coli strain MJF612 was used as a host for E. coli MscL (MscL), K55T E. coli MscL (K55T MscL), B. subtilis MscL (Bsub MscL), S. aureus MscL (Sau MscL) and E. coli MscS (MscS) constructs in the pB10d expression vector. Overnight cultures were grown in CphM plus 100 μg ml −1 ampicillin in a shaker incubator at 37 °C and rotated at 250 cycles per min. The next morning, cultures were diluted to 1:60 in the same media and grown for 30 min before inducing expression with 1 mM IPTG. After 1 h of induction, all cultures were adjusted to an OD 600 of 0.1. The cultures were then diluted 1:3 into pre-warmed CphM plus 100 μg ml −1 ampicillin plus the antibiotic being tested. Cultures were loaded in 96-well plates (180 μl per well) in 7 replicates; plates were sealed with a breathable film for 96-well plates to avoid evaporation, wrapped in foil and incubated at 37 °C for 16 h without shaking. The OD 600 of the cultures was measured using a Multiskan Ascent (Thermo Scientific Inc., Waltham, MA, USA). The antibiotics were diluted to their final concentration from the following stock solutions: viomycin sulphate (USP, Rockville, MD, USA) 5 mM in H 2 O; nifuroxazide (Sigma, St Louis, MO, USA) 5 mM in DMSO; dihydrostreptomycin (Sigma) and spectinomycin (Sigma) 50 mM in H 2 O. Viability experiments Cultures were started from single colonies and grown in Lennox Broth (LB) medium (Fisher Scientific, Pittsburgh, PA, USA) plus ampicillin (100 μg ml −1 ). Overnight cultures were diluted 1:40 in the same media and grown to an OD 600 of 0.2. Cell lines with plasmids were then induced for 30 min to 1 h with 1 mM IPTG. After adjusting all cultures to an OD 600 =0.4, cultures were serially diluted from 10 3 to 10 6 in LB and liquid drops of 5 μl of each dilution were placed on pre-warmed LB plates containing 1 mM IPTG and either no drugs, or varying amounts of dihydrostreptomycin. Colony-forming units were counted to determine cell viability. Typical values for the 100% values were 6–8 × 10 7 colony-forming units. Electrophysiology E. coli giant spheroplasts were generated as previously described [23] from MJF612 strain expressing the K55T MscL mutant in trans . Patch clamp experiments were performed in the inside-out configuration, at room temperature under symmetrical conditions using a buffer consisting of 200 mM KCl, 90 mM MgCl 2 , 10 mM CaCl 2 and 5 mM HEPES adjusted to pH 6.0. Patches were excised, and recordings were performed at 20 mV (for simplicity the patch traces openings are shown upward). Data were acquired at a sampling rate of 20 kHz with 10 kHz filtration using an AxoPatch 200B amplifier (Molecular Devices, Sunnyvale, CA, USA). A piezoelectric pressure transducer (World Precision Instruments, Sarasota, FL, USA) was used to measure the pressure throughout the experiments. Glass pipettes were backfilled with the antibiotic, with the tip containing patch buffer without the drugs. Traces taken right after the patch-seal formation were used as controls for each experiment. Only patches that form seals within 3 min of backfilling the pipette were used, and MscL response to pressure was measured immediately after forming the patch. Three consecutive measurements were taken for the control at the first time point, and MscL sensitivity within the patch was tested subsequently every 20 min. Potassium flux experiments The MJF612 strain was used for the K + flux experiments [17] either carrying an empty vector or expressing WT MscL. Overnight cultures were grown from a single colony in K10 media consisting of 46 mM Na 2 HPO 4 , 23 mM NaH 2 PO 4 , 8 mM (NH 4 ) 2 SO 4 , 10 mM KCl and 100 mM NaCl, supplemented with 0.4 mM MgSO 4 , 3 μM thiamine, 6 μM iron, 0.04% glucose plus 100 μg ml −1 ampicillin. The next morning, cultures were diluted 1:50 in the same media; when they reached an OD 600 =0.2, they were induced for 1 h at 37 °C. The cultures were then split in two: mock (no drug added) and with 82 μM or 140 μM dihydrostreptomycin. The final OD 600 was taken and the amount of cells to be used was calculated, adjusting for OD. Typical OD values ranged from 0.47 to 0.67, and approximately 1–1.5 ml of the cultures were then passed through a 0.45-μm filter and washed with 3 ml of K0 media (K10 with the KCl replaced by NaCl), of the same osmolarity and no supplements or ampicillin. The filters were placed in 100-ml plastic beakers and then dried in an oven at 80 °C overnight covered with foil. The next morning, 3 ml of double-distilled water were added to each filter and K + levels were read using a flame photometer after a standard curve was established. Typical values ranged from 90 to 140 mM, and about 50–70 mM for the streptomycin-treated bacteria expressing MscL. Glutamate assay The MJF612 strain was used for the K + flux experiments [17] either carrying an empty vector or expressing WT MscL. Overnight cultures were grown from a single colony in K10 media consisting of 46 mM Na 2 HPO 4 , 23 mM NaH 2 PO 4 , 8 mM (NH 4 ) 2 SO 4 , 10 mM KCl and 100 mM NaCl, supplemented with 0.4 mM MgSO 4 , 3 μM thiamine, 6 μM iron, 0.04% glucose plus 100 μg ml −1 ampicillin. The next morning, cultures were diluted 1:50 in the same media; when they reached an OD 600 =0.2, they were induced for 1 h at 37 °C. The cultures were then split in two: mock (no drug added) and with 82 μM dihydrostreptomycin. The final OD 600 of the cultures was recorded and 15 ml of each sample was pelleted, the supernatant removed and immediately frozen down to −80 °C. Samples were resuspended in K0 media (no supplements) adjusting volume for final OD 600 . Glutamate measurements were performed using the EnzyChrom Glutamate Assay Kit (BioAssay Systems, Hayward, CA, USA) according to the manufacturer’s instructions. I.I. developed the HTS assay and performed the screen with the assistance, guidance and help of S.W. and under the supervision of B.P. R.W. performed the in vivo physiological and ion flux assays. I.I. performed electrophysiology, and P.B. initially conceived and supervised the project. All authors contributed intellectually to the project and to the writing of the manuscript. How to cite this article: Iscla, I. et al. Streptomycin potency is dependent on MscL channel expression. Nat. Commun. 5:4891 doi: 10.1038/ncomms5891 (2014).